Ligand-specific deactivation time course of GluN1/GluN2D NMDA receptors N -methyl- D -aspartate (NMDA) receptors belong to the family of ionotropic glutamate receptors that mediate a majority of excitatory synaptic transmission. One unique property of GluN1/GluN2D NMDA receptors is an unusually prolonged deactivation time course following the removal of L -glutamate. Here we show, using x-ray crystallography and electrophysiology, that the deactivation time course of GluN1/GluN2D receptors is influenced by the conformational variability of the ligand-binding domain (LBD) as well as the structure of the activating ligand. L -glutamate and L -CCG-IV induce significantly slower deactivation time courses compared with other agonists. Crystal structures of the isolated GluN2D LBD in complex with various ligands reveal that the binding of L -glutamate induces a unique conformation at the backside of the ligand-binding site in proximity to the region at which the transmembrane domain would be located in the intact receptors. These data suggest that the activity of the GluN1/GluN2D NMDA receptor is controlled distinctively by the endogenous neurotransmitter L -glutamate. A majority of communication between neurons is mediated by release and reception of neurotransmitters at the synapse. On binding to neurotransmitters, ligand-gated ion channels generate postsynaptic currents that serve as neuronal signals. This neurotransmission dictates the strength of neuronal interactions, and is a major currency for brain development and function. In the mammalian brain, the strength and time course of L -glutamate-mediated excitatory postsynaptic currents are determined by the functional properties of ionotropic glutamate receptors (iGluRs), which can be classified into three pharmacological and gene families, including α-amino-3-hydroxy-5-methyl-4-propionic acid (AMPA), kainate and N -methyl- D -aspartate (NMDA) receptors [1] , [2] . NMDA receptors deactivate significantly more slowly than non-NMDA receptors, thus comprising the slow component of excitatory postsynaptic signals [3] , [4] . NMDA receptors are tetrameric ion channels composed of two GluN1 subunits and two GluN2 subunits, and are unique among the iGluR family members in that activation requires concurrent binding of glycine and L -glutamate to the GluN1 and GluN2 subunits, respectively [1] , [2] . NMDA receptor subunits possess a modular design and are composed of an amino-terminal domain (ATD), a ligand-binding domain (LBD), a transmembrane domain that forms the ion channel pore and an intracellular carboxyl-terminal domain. The recent crystallographic study on the full-length homomeric GluA2 receptor has revealed the overall architecture of domain organization of a tetrameric subunit arrangement for AMPA receptors [5] . In contrast, structure–function studies of NMDA receptors have lagged behind AMPA receptors, primarily because of experimental complexities stemming from the heteromeric assembly of the GluN1 and GluN2 subunits. Nevertheless, structural insights into NMDA receptor function have been gained through recent crystallographic studies on the LBDs [6] , [7] , [8] , [9] . The most extensive studies have been conducted on the LBDs of the GluN1/GluN2A [7] and the GluN3A and GluN3B subunits [9] , revealing a bilobed clamshell-like architecture composed of domain-1 (D1) and domain-2 (D2), with a ligand-binding pocket at the D1–D2 cleft, similar to the structure of the non-NMDA receptor LBDs [6] , [7] , [8] . However, there are substantial differences in how conformational changes couple to gating of the ion channels between AMPA and NMDA receptors, indicating that the physicochemical properties of the LBDs may depend on the subunit [10] . The four distinct GluN2 subunits (GluN2A–GluN2D) provide the functional and pharmacological diversity of NMDA receptors, including differences in potency and deactivation time course [1] , [11] . NMDA receptors that contain the GluN2D subunit have ~ 40-fold longer deactivation time course compared with receptors containing GluN2A [12] , [13] . The unique properties of the GluN2D-containing NMDA receptors are considered important both for early brain development as well as function of neurons specifically expressing the GluN2D subunits in the mature brain [14] , [15] , [16] . Several lines of investigation have identified factors that regulate deactivation time course in NMDA receptors. For example, some studies have suggested that the ligand association and dissociation rates at the LBDs are the primary determinants of the deactivation time course of neuronal and GluN2A-containing NMDA receptors, as well as AMPA and kainate receptors [7] , [17] , [18] , [19] . Furthermore, recent studies have shown that the GluN2 ATD and a linker between the ATD and the LBD (ATD–D1 linker) influence deactivation time course [20] , [21] , indicating that the ATD exerts significant control over deactivation. Previous single-channel studies have shown that the deactivation time course of macroscopic currents of NMDA receptors is dependent on channel burst length [4] , which has been shown to depend on a series of rate constants that describe NMDA receptor gating and differ according to the type of GluN2 subunit present in the receptor [13] , [21] , [22] , [23] . In this study, we measure the deactivation time course of recombinant GluN1/GluN2D receptor currents induced by a range of agonists. The data show that L -glutamate elicits a much slower deactivation time course compared with other excitatory amino acids. Crystallographic studies of the isolated GluN2D LBD monomer show a unique conformation around the hinge and D2 domains of the bilobed clamshell when complexed with L -glutamate compared with other ligands. Moreover, structure-based mutagenesis suggests that the differences in amino acids between the GluN2A and GluN2D LBDs may distinctively influence the time course of deactivation. These data are consistent with the idea that the unique conformation of the L -glutamate-bound LBD may underlie the unusually slow deactivation time course for L -glutamate in the GluN1/GluN2D receptors. Linear non- L -glutamate agonists evoke rapid GluN2D deactivation To assess the dependence of the deactivation time course of GluN1/GluN2D NMDA receptors on the structure of activating ligands, we recorded whole-cell responses under voltage clamp from HEK cells expressing recombinant GluN1/GluN2D and compared the response time courses of a series of glutamate and aspartate analogues. The coagonist glycine was present in all solutions (0.05 mM), and current responses were evoked with a 1-s pulse of 1-mM agonist. Following a 1-s pulse of 1-mM L -glutamate, the GluN1/GluN2D receptors deactivated slowly with a dual exponential time course with time constants of τ Fast =930±100 ms and τ Slow =3,200±240 ms ( n =30; Fig. 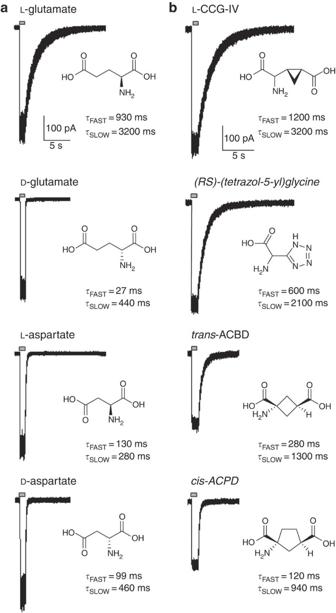Figure 1: Deactivation time course is dependent on ligand structure. HEK cells were activated under voltage clamp by maximally effective concentrations of various linear agonists (a;L-glutamate,D-glutamate,L-aspartate andD-aspartate) and cyclic agonists (b;L-CCG-IV,trans-ACBD, (RS)-(tetrazol-5-yl)glycine andcis-ACPD) applied for 1 s; all solutions contained 0.05-mM glycine.L-glutamate andL-CCG-IV evoked the slowest deactivation time courses of the ligands examined. All other linear and cyclic agonists evoked significantly more rapid deactivation time courses compared withL-glutamate orL-CCG-IV. The deactivation time constants are given as the mean of 5–26 cells. 1a ; Table 1 ), as previously described [12] , [13] , [21] . Interestingly, the stereoisomer D -glutamate caused the receptor to deactivate much more rapidly, with time constants of τ Fast =27±2.4 ms and τ Slow =440±120 ms ( n =12; Fig. 1a ; Table 1 ). Figure 1: Deactivation time course is dependent on ligand structure. HEK cells were activated under voltage clamp by maximally effective concentrations of various linear agonists ( a ; L -glutamate, D -glutamate, L -aspartate and D -aspartate) and cyclic agonists ( b ; L -CCG-IV, trans -ACBD, ( RS )-(tetrazol-5-yl)glycine and cis -ACPD) applied for 1 s; all solutions contained 0.05-mM glycine. L -glutamate and L -CCG-IV evoked the slowest deactivation time courses of the ligands examined. All other linear and cyclic agonists evoked significantly more rapid deactivation time courses compared with L -glutamate or L -CCG-IV. The deactivation time constants are given as the mean of 5–26 cells. Full size image Table 1 Deactivation time course of GluN2D- and GluN2A-containing receptors. Full size table We subsequently assessed deactivation time course for other agonists. The glutamate analogue L -homocysteate, which has been detected in the brain and may function as an endogenous neurotransmitter [24] , [25] , [26] , [27] , also caused the GluN1/GluN2D receptor to deactivate much more rapidly than L -glutamate ( Table 1 ). L -aspartate ( τ Fast =130±10 ms; τ Slow =280±25 ms; n =8) and D -aspartate ( τ Fast =99±8.3 ms; τ Slow =460±100 ms; n =7) had similar deactivation time constants, both of which are faster than L -glutamate ( Fig. 1a ; Table 1 ). This suggests that any GluN2D-containing NMDA receptor at synapses at which aspartate participates as a primary neurotransmitter may deactivate more rapidly than synapses at which L -glutamate is released [28] , [29] , [30] , [31] , [32] . Cyclic agonists evoke slow GluN2D deactivation Several compounds with conformationally constrained rings function as partial agonists of NMDA receptors ( Table 1 , Supplementary Table S1 ), in some cases with higher potency (that is, lower half maximal effective concentration, or EC 50 ) compared with L -glutamate [33] . We tested whether these compounds could evoke a slower deactivation time course than L -glutamate ( Fig. 1b ). Agonists (plus 0.05-mM glycine) were applied for 1 s at concentrations of 0.1–1 mM to HEK cells expressing GluN1/GluN2D. The most potent cyclic ligand L -CCG-IV, with an EC 50 value (36 nM) that was tenfold lower than L -glutamate, deactivated with a time course that was significantly different ( P <0.05; analysis of variance (ANOVA)) from all ligands except L -glutamate ( τ Fast =1,200±290 ms and τ Slow =3,200±600 ms). trans -ACBD, with a similar potency to L -glutamate, deactivated significantly faster than L -glutamate, with time constants of τ Fast =280±69 ms and τ Slow =1,300±320 ms ( n =5; Fig. 1b , Table 1 ; ANOVA). Relationship of GluN1/GluN2D deactivation and agonist potency Previous studies have demonstrated that the deactivation time course is correlated with the ligand EC 50 for AMPA receptors [34] . 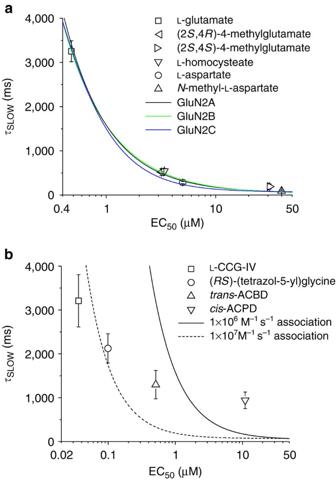Figure 2: The relationship between deactivation and EC50. (a) The relationship between the experimentally determinedτSlowand the EC50value for the steady-state response is shown for linear ligands for whichτSlowcontributes >10% to the deactivation time course (L-glutamate,L-homocysteate,L-aspartate, NMLA, (2S,4R)-4-methylglutamate and (2S,4S)-4-methylglutamate). Superimposed on these data are simulated response properties from modified NMDA receptor-gating models for GluN1/GluN2A, GluN1/GluN2B and GluN1/GluN2C23,35,36adapted forL-glutamate-activated GluN1/GluN2D receptors by removal of the desensitized states (seeMethodsandSupplementary Fig. S1). We first determined association and dissociation rate constants that yielded a steady-state EC50and deactivation time constant similar to that measured forL-glutamate-activated GluN1/GluN2D. We subsequently simulated the responses of each adapted model using an association rate (b+) of 1.0×106M−1s−1. The dissociation rates (b−) were varied between 0.1 and 100 s−1, while holding the gating rates constant. The solid lines show the relationship between the EC50value and τ-deactivation for each adapted model. (b) The relationship between experimentally determined EC50values andτSlowfor the cyclic ligands is shown. Superimposed on this plot is the relationship between τ-deactivation and the EC50value predicted forL-glutamate activation of the GluN1/GluN2A-adapted model as dissociation rates vary between 0.5 and 100 s−1(solid line). Simulations using the same rate constants and a faster association rate (1.0×107M−1s−1) are shown (broken line; gating rates held constant). The faster association rates provided a better prediction of theτSlowofL-CCG-IV and (RS)-(tetrazol-5-yl)glycine, but did not predict the deactivation time courses oftrans-ACBD andcis-ACPC. Figure 2a shows the relationship between experimentally determined EC 50 and τ Slow for GluN1/GluN2D receptors activated by linear ligands for which τ Slow accounted for >10% of the deactivation time course. Although it would be informative to evaluate the relationship between deactivation, agonist EC 50 and agonist dissociation rate using models of NMDA receptor gating, a kinetic scheme that can reproduce the low open probability, rapid rise time, slow deactivation, absence of desensitization, high glutamate potency and single-channel properties of GluN1/GluN2D is not available. We therefore utilized modified models of GluN1/GluN2A, GluN1/GluN2B and GluN1/GluN2C receptor function in which desensitization steps were removed and binding states were altered [23] , [35] , [36] to explore the relationship between τ-deactivation and EC 50 values as the dissociation rate varied (see Methods and Supplementary Fig. S1 ). Whereas these adapted models only approximately predict the properties of GluN1/GluN2D they nevertheless provide insight into the relationship between the time course for deactivation and the EC 50 value for NMDA receptors as the glutamate dissociation rate is varied. Figure 2a shows that this relationship for glutamate superimposed on experimentally determined τ Slow and EC 50 for linear agonists that have a sufficiently large slow component (>10%) of deactivation that allows reliable determinations of τ Slow . Although gating rates almost certainly vary among ligands, these measured parameters lie close to the predicted curve for L -glutamate. However, these models do not predict measured response properties of cyclic ligands, which have fewer conformational degrees of freedom than linear agonists and the actions of which may be described by rates that differ substantially from L -glutamate ( Fig. 2b ). Whereas these data show how the experimentally determined τ Slow relates to the EC 50 for linear ligands activating GluN1/GluN2D receptors, the adapted models do not predict a fast component of deactivation comparable to that determined experimentally for GluN1/GluN2D receptors. At present, factors that control the magnitude or relative contribution of the faster time constant describing the deactivation time course of GluN1/GluN2D receptors remain unknown. Figure 2: The relationship between deactivation and EC 50 . ( a ) The relationship between the experimentally determined τ Slow and the EC 50 value for the steady-state response is shown for linear ligands for which τ Slow contributes >10% to the deactivation time course ( L -glutamate, L -homocysteate, L -aspartate, NMLA, (2 S ,4 R )-4-methylglutamate and (2 S ,4 S )-4-methylglutamate). Superimposed on these data are simulated response properties from modified NMDA receptor-gating models for GluN1/GluN2A, GluN1/GluN2B and GluN1/GluN2C [23] , [35] , [36] adapted for L -glutamate-activated GluN1/GluN2D receptors by removal of the desensitized states (see Methods and Supplementary Fig. S1 ). We first determined association and dissociation rate constants that yielded a steady-state EC 50 and deactivation time constant similar to that measured for L -glutamate-activated GluN1/GluN2D. We subsequently simulated the responses of each adapted model using an association rate ( b + ) of 1.0×10 6 M −1 s −1 . The dissociation rates ( b − ) were varied between 0.1 and 100 s −1 , while holding the gating rates constant. The solid lines show the relationship between the EC 50 value and τ-deactivation for each adapted model. ( b ) The relationship between experimentally determined EC 50 values and τ Slow for the cyclic ligands is shown. Superimposed on this plot is the relationship between τ-deactivation and the EC 50 value predicted for L -glutamate activation of the GluN1/GluN2A-adapted model as dissociation rates vary between 0.5 and 100 s −1 (solid line). Simulations using the same rate constants and a faster association rate (1.0×10 7 M −1 s −1 ) are shown (broken line; gating rates held constant). The faster association rates provided a better prediction of the τ Slow of L -CCG-IV and ( RS )-(tetrazol-5-yl)glycine, but did not predict the deactivation time courses of trans -ACBD and cis -ACPC. Full size image GluN1/GluN2D deactivation is not influenced by desensitization Previous studies have demonstrated that even brief pulses of agonist can induce some desensitization of GluN1/GluN2A NMDA receptors [37] . We cannot detect any desensitization of GluN1/GluN2D macroscopic current response in whole-cell recordings. Nevertheless, we used a paired-pulse paradigm on excised patches containing GluN1/GluN2D receptors to evaluate whether some receptors might enter a desensitized state from which they recover during deactivation. The peak current amplitude and deactivation time course of GluN1/GluN2D receptors seem to be uninfluenced by desensitization using a paired-pulse protocol following a 2-ms or 4-s application of 1-mM L -glutamate and 0.05-mM glycine to excised outside-out patches ( n =8; Supplementary Fig. S2 ). Whereas it is possible that the receptor desensitizes more rapidly than can be detected (that is, within a few microseconds), we do not observe any effect of desensitization on the deactivation time course ( Supplementary Fig. S2 ). Crystal structures of GluN2D LBD To evaluate the idea that GluN2D may adopt unique agonist-dependent conformations that influence the deactivation time course, we used X-ray crystallography to explore the structures of the isolated GluN2D LBD monomer in complex with four agonists: L -glutamate, D -glutamate, L -aspartate and NMDA. The crystals showed X-ray diffractions higher than 1.9 Å ( Supplementary Table S2 ), which resulted in structures with unambiguous electron densities for proteins, ligands and water molecules. The GluN2D LBD has a bilobed clamshell-like architecture composed of domains D1 and D2 ( Fig. 3a,b ), similar to that observed in the previously solved GluN2A LBD structure [7] . The GluN2A and GluN2D structures in complex with L -glutamate can be superimposed to one another with root mean square deviation of 0.88 Å over 240 out of 285 possible Cα positions ( Fig. 3c ). However, there are two regions in the clamshell structures that are distinct from one another: the conformation of the loop at the backside of the ligand-binding site ('hinge loop'; Fig. 3c ), and loop-1 tethered to the protein core by two disulphide bonds in domain D1 ( Fig. 3a , Supplementary Fig. S3 ). Interestingly, the structures of GluN2D in complex with NMDA, L -aspartate and D -glutamate show similarity to GluN2A at the hinge loop ( Fig. 3d ), raising the possibility that ligands that show rapid deactivation from GluN2D produce a conformation similar to that of GluN2A. 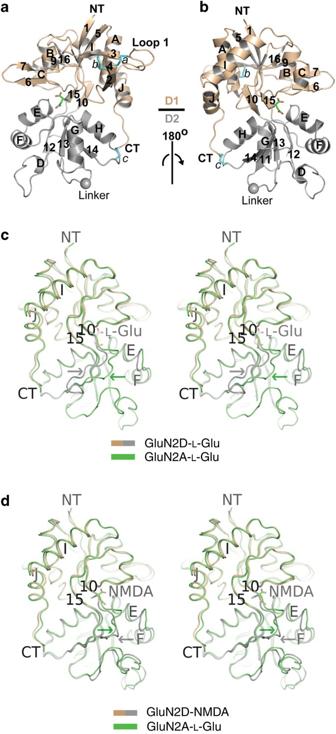Figure 3: Crystal structure of GluN2D LBD. (a,b) Overall structure of the bilobed GluN2D LBD in complex with NMDA (green sticks) is shown with the N terminus (NT) and C terminus (CT) on top and bottom, respectively. Ligands such as NMDA bind to the interdomain cleft between domain 1 (D1; wheat) and domain 2 (D2; light grey). Three disulphide bonds (a–c; cyan sticks) are formed between the following cysteine pairs: Cys452 and Cys490 (a), Cys459 and Cys481 (b), and Cys770 and Cys825 (c). The sphere indicated as 'linker' is the Cα of glycine in the Gly and Thr residues that replace the transmembrane domains. (c) Structural comparison betweenL-glutamate bound to GluN2D (wheat and light grey) and GluN2A (PDB code:2A5S, green) in stereoview. The superposition shows the divergent region, the hinge loop (green arrow: GluN2A and grey arrow: GluN2D), proximal to helices-E and -F, and strands 15 and 16. The orientation of the structures is the same as that inb. (d) Structural comparison between NMDA-bound GluN2D (wheat and light grey) andL-glutamate-bound GluN2A (green) in stereoview. The superposition shows a similarity in orientation of hinge loops (arrows) between GluN2A and GluN2D. The root mean square deviation of superposition is 1.10 Å over 263 Cα positions. Disulphide bonds are omitted for clarity incandd. Figure 3: Crystal structure of GluN2D LBD. ( a , b ) Overall structure of the bilobed GluN2D LBD in complex with NMDA (green sticks) is shown with the N terminus (NT) and C terminus (CT) on top and bottom, respectively. Ligands such as NMDA bind to the interdomain cleft between domain 1 (D1; wheat) and domain 2 (D2; light grey). Three disulphide bonds (a–c; cyan sticks) are formed between the following cysteine pairs: Cys452 and Cys490 (a), Cys459 and Cys481 (b), and Cys770 and Cys825 (c). The sphere indicated as 'linker' is the Cα of glycine in the Gly and Thr residues that replace the transmembrane domains. ( c ) Structural comparison between L -glutamate bound to GluN2D (wheat and light grey) and GluN2A (PDB code: 2A5S , green) in stereoview. The superposition shows the divergent region, the hinge loop (green arrow: GluN2A and grey arrow: GluN2D), proximal to helices-E and -F, and strands 15 and 16. The orientation of the structures is the same as that in b . ( d ) Structural comparison between NMDA-bound GluN2D (wheat and light grey) and L -glutamate-bound GluN2A (green) in stereoview. The superposition shows a similarity in orientation of hinge loops (arrows) between GluN2A and GluN2D. The root mean square deviation of superposition is 1.10 Å over 263 Cα positions. Disulphide bonds are omitted for clarity in c and d . Full size image A striking feature of the GluN2D LBD structures in complex with various ligands is the considerable difference in the conformation of the 'hinge loop' between the L -glutamate-bound form and all the other forms ( Fig. 4a ). The loop spans eight residues from Ile775 to Ala782, with a large difference in Cα positions ranging from ~1.4 to 9.8 Å between the L -glutamate-bound structures and the other three structures ( Fig. 4 ). The hinge loops in the L -aspartate-, D -glutamate- and NMDA-bound structures have similar conformations and interact with a structural motif containing helix-E and -F through hydrophobic interactions involving Tyr723, Val780 and Phe781 ( Fig. 4d ). This particular orientation of the hinge loop stabilizes the interaction with the structural motif containing helix-D and loop-D, which is located in proximity to the Gly–Thr linker, through hydrophobic interactions mediated by a cluster of nonpolar residues, including Ile558, Leu690, Val780 and Phe781 ( Fig. 4d ). All of the above interactions tie the hinge loop, helix-E and -F, and helix-D and loop-D into one unit ( Fig. 4d ). In contrast, in the L -glutamate-bound structure, these interactions are absent because of a large conformational difference in the hinge loop; instead of helix-E and -F, the hinge loop is tied to helix-H through a nonpolar interaction between Val780 and Ala757 ( Fig. 4e ). Furthermore, in the L -glutamate-bound structure, helix-D and loop-D are disordered, likely, because the hinge loop in the L -glutamate-bound conformation may not be suitable to form an interaction with loop-D and may not be able to lock the conformation of loop-D. 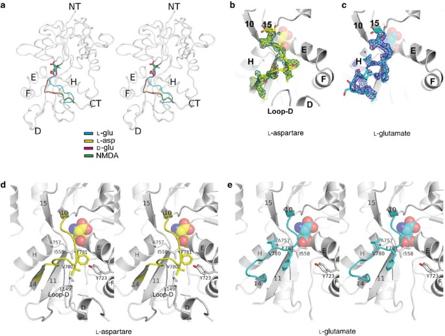Figure 4: Conformational variability at the clamshell hinge. (a) Stereoview of the overall structures of the GluN2D LBD in complex with various ligands. The structural superposition reveals a distinct conformation of hinge loops (coloured loops) between theL-glutamate-bound form (cyan) and all the other forms (L-aspartate, yellow;D-glutamate, magenta; and NMDA, green). Ligands are shown as sticks. (b,c) Fo-Fc omits electron density of the hinge loop contoured at 2.8σ for theL-aspartate- (b) andL-glutamate-bound (c) structures. The residues are well ordered, except for a portion of Lys779, as shown by a breakage at the electron density map. (d,e) Different modes of interactions between the hinge loop and helices-E-F or helix-H in theL-aspartate-bound (d) andL-glutamate-bound (e) structures in stereoview. The loop that contains Leu690 in theL-aspartate-bound structure (loop-D) and helix-D are disordered in theL-glutamate-bound structure. Ligands are shown as spheres. Residues on the hinge loops are coloured as yellow and cyan forL-aspartate-bound andL-glutamate-bound structures, respectively. Residues proximal to the hinge loop are in white. Figure 4: Conformational variability at the clamshell hinge. ( a ) Stereoview of the overall structures of the GluN2D LBD in complex with various ligands. The structural superposition reveals a distinct conformation of hinge loops (coloured loops) between the L -glutamate-bound form (cyan) and all the other forms ( L -aspartate, yellow; D -glutamate, magenta; and NMDA, green). Ligands are shown as sticks. ( b , c ) Fo-Fc omits electron density of the hinge loop contoured at 2.8σ for the L -aspartate- ( b ) and L -glutamate-bound ( c ) structures. The residues are well ordered, except for a portion of Lys779, as shown by a breakage at the electron density map. ( d , e ) Different modes of interactions between the hinge loop and helices-E-F or helix-H in the L -aspartate-bound ( d ) and L -glutamate-bound ( e ) structures in stereoview. The loop that contains Leu690 in the L -aspartate-bound structure (loop-D) and helix-D are disordered in the L -glutamate-bound structure. Ligands are shown as spheres. Residues on the hinge loops are coloured as yellow and cyan for L -aspartate-bound and L -glutamate-bound structures, respectively. Residues proximal to the hinge loop are in white. Full size image The local conformational change described above is unlikely to reflect crystallographic artefacts for two reasons. First, all of the crystals in complex with four ligands have been grown in the same condition and are isomorphous to each other; therefore, no chemical factor favours one conformation over another. Second, no crystal contact forces the hinge loop, helix-D, -E and -F, and loop-D into the observed conformations. Thus, the crystal packing around the region is sufficiently 'loose' to allow conformational change within the crystal lattice. Finally, soaking the GluN2D LBD- L -aspartate crystals against a buffer containing L -glutamate can change the hinge conformation to that observed in the GluN2D LBD- L -glutamate cocrystal structure. The current study is the first that structurally shows the binding pattern of NMDA to GluN2 receptors. Therefore, the molecular determinants defining the selectivity for the agonist NMDA can now be visualized ( Fig. 5 ). Electron density for all ligands, situated at the clamshell cleft between D1 and D2, is visible owing to the high-resolution X-ray diffraction data ( Fig. 5a–d ). The ligands tested in this study bind to GluN2D through direct polar interactions involving the main-chain oxygens and nitrogens of Ser536, Thr538, Arg543, Ser714 and Thr715, which are conserved in the binding of L -glutamate to GluN2A [7] . In addition to the polar interactions, the binding of NMDA involves displacement of a water molecule (W in Fig. 5a–d ) by the N -methyl group, the placement of which is favoured by the surrounding hydrophobic residues, Tyr755 and Val759. The equivalent residues for Tyr755 in AMPA and kainate receptors are leucine and methionine, respectively, pointing away from the binding pocket ( Fig. 5e ). The corresponding residues for Val759 are methionine in AMPA receptors and threonine in kainate receptors, which are more hydrophilic ( Fig. 5e ). Furthermore, Asp756 folds away from the binding pocket so that its β-carboxyl group does not interfere with the placement of the N -methyl group of NMDA. The aspartate residue at the 756 position is conserved among the subunits of NMDA receptors. In non-NMDA receptors, the equivalent residue of Asp756 is glutamate, the longer side chain of which would collide with the N -methyl group and disallow the placement of an NMDA molecule in their binding pockets. 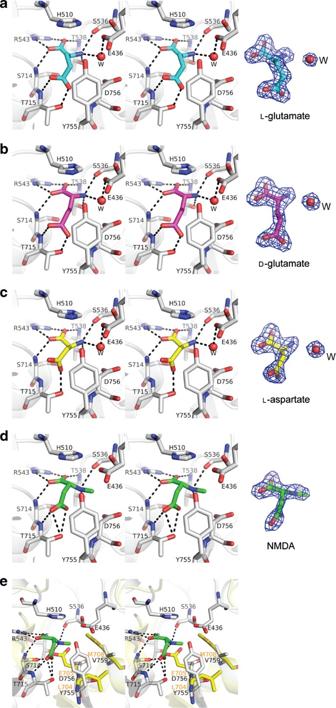Figure 5: Agonist-binding site of GluN2D and determinants for NMDA specificity. (a–d) All of the ligands tested in this study bind in the interdomain cleft between domains D1 and D2. Shown here are stereoviews of the ligand-binding site of GluN2D in complex withL-glutamate (a; cyan),D-glutamate (b; magenta),L-aspartate (c; yellow) and NMDA (d; green). A water molecule (W) present in theL-glutamate-,D-glutamate- andL-aspartate-binding pocket is represented by a red sphere. Shown on the right hand side ofa–din blue mesh are Fo−Fc omit difference Fourier maps for the ligands and the attached water molecule contoured at 4σ. (e) Structures of the GluN2D LBD (grey) and GluA2 LBD (PDB code1FTJ; yellow) are superimposed to one another to show unfavourable placement of NMDA molecule (green) in non-NMDA receptors. Corresponding residues of GluN2D Tyr755, Asp756 and Val759 in GluA2 are Leu704, Glu705 and Met708 (yellow), respectively. The placement of theN-methyl group of NMDA is favoured in the GluN2 subunit because of the hydrophobic environment created by Tyr755 and Val759, and because of the location of the Asp756 side chain away from the pocket. In AMPA receptors, the equivalent residue to Asp756 is glutamate (Glu705), the longer side chain of which would collide with theN-methyl group. The binding is also disfavoured because of replacement of Val759 with methionine, which makes the binding pocket less hydrophobic. Figure 5: Agonist-binding site of GluN2D and determinants for NMDA specificity. ( a – d ) All of the ligands tested in this study bind in the interdomain cleft between domains D1 and D2. Shown here are stereoviews of the ligand-binding site of GluN2D in complex with L -glutamate ( a ; cyan), D -glutamate ( b ; magenta), L -aspartate ( c ; yellow) and NMDA ( d ; green). A water molecule (W) present in the L -glutamate-, D -glutamate- and L -aspartate-binding pocket is represented by a red sphere. Shown on the right hand side of a – d in blue mesh are Fo−Fc omit difference Fourier maps for the ligands and the attached water molecule contoured at 4σ. ( e ) Structures of the GluN2D LBD (grey) and GluA2 LBD (PDB code 1FTJ ; yellow) are superimposed to one another to show unfavourable placement of NMDA molecule (green) in non-NMDA receptors. Corresponding residues of GluN2D Tyr755, Asp756 and Val759 in GluA2 are Leu704, Glu705 and Met708 (yellow), respectively. The placement of the N -methyl group of NMDA is favoured in the GluN2 subunit because of the hydrophobic environment created by Tyr755 and Val759, and because of the location of the Asp756 side chain away from the pocket. In AMPA receptors, the equivalent residue to Asp756 is glutamate (Glu705), the longer side chain of which would collide with the N -methyl group. The binding is also disfavoured because of replacement of Val759 with methionine, which makes the binding pocket less hydrophobic. Full size image Molecular correlates of GluN1/GluN2D deactivation time course Our data demonstrate that the deactivation time course of the GluN1/GluN2D receptors differs markedly between currents evoked by L -glutamate and other linear agonists. Surprisingly, the ligand dependence on the relative amplitudes of the two time constants (fast and slow) describing deactivation time course observed in the GluN1/GluN2D receptors is largely absent in the GluN1/GluN2A receptors ( Table 1 ). Furthermore, the conformation of the GluN2D LBD structure is dependent on the agonist, differing when in complex with L -glutamate compared with D -glutamate, L -aspartate and NMDA. These observations imply that the ligands induce conformational changes within the GluN2D LBD, which may be the contributing factors in the regulation of the deactivation time course following agonist removal. To test this hypothesis, we measured the deactivation time courses of D - and L -glutamate-induced currents from chimeric NMDA receptors ( Fig. 6 ). We chose to make chimeric receptors between GluN2A and GluN2D because GluN1/GluN2A receptors deactivate more rapidly than GluN1/GluN2D receptors when activated by L -glutamate, providing the greatest difference in deactivation time course among all GluN2 subunits. In addition, crystal structures of the L -glutamate-bound GluN2A LBD have been previously described [7] , allowing design of chimeric receptors that minimally perturb the overall subunit architecture. 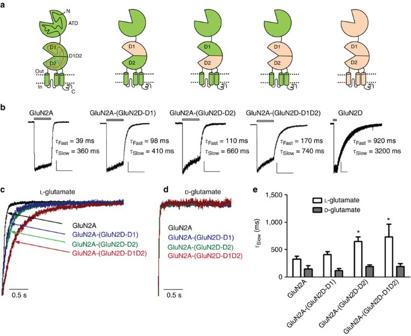Figure 6: Assessment of molecular correlates of GluN2D deactivation. (a) Cartoons of the wild-type and chimeric receptors are given, with GluN2A in green and GluN2D in wheat. (b)L-glutamate (1 mM) was applied rapidly to transfected HEK cells for 1 s (grey bars); 0.05-mM glycine was present in all solutions. Inserting portions or the full GluN2D–D1D2 LBD increased the fast and slow time constants describing the deactivation time course compared with the time constants of GluN1/GluN2A. The horizontal scale bar represents 2 s for all traces, and the vertical scale bar represents ~200 pA for all traces. (c) Normalized current traces of the deactivation time courses of GluN2A and chimeric receptors following removal ofL-glutamate. (d) Normalized current traces of GluN2A and chimeric receptors following the removal ofD-glutamate. The deactivation time course following removal ofD-glutamate did not significantly lengthen for any chimeric receptor. (e) The slow deactivation time constant (τSlow) of GluN2A and the chimeric receptors is given forL-glutamate (white bars) andD-glutamate (grey bars). Bars are given in mean±s.e.m. *P<0.05 when compared with the deactivation time course of GluN1/GluN2A activated byL-glutamate and analysed by one-way ANOVA with Tukey'spost hoctest. Figure 6: Assessment of molecular correlates of GluN2D deactivation. ( a ) Cartoons of the wild-type and chimeric receptors are given, with GluN2A in green and GluN2D in wheat. ( b ) L -glutamate (1 mM) was applied rapidly to transfected HEK cells for 1 s (grey bars); 0.05-mM glycine was present in all solutions. Inserting portions or the full GluN2D–D1D2 LBD increased the fast and slow time constants describing the deactivation time course compared with the time constants of GluN1/GluN2A. The horizontal scale bar represents 2 s for all traces, and the vertical scale bar represents ~200 pA for all traces. ( c ) Normalized current traces of the deactivation time courses of GluN2A and chimeric receptors following removal of L -glutamate. ( d ) Normalized current traces of GluN2A and chimeric receptors following the removal of D -glutamate. The deactivation time course following removal of D -glutamate did not significantly lengthen for any chimeric receptor. ( e ) The slow deactivation time constant ( τ Slow ) of GluN2A and the chimeric receptors is given for L -glutamate (white bars) and D -glutamate (grey bars). Bars are given in mean±s.e.m. * P <0.05 when compared with the deactivation time course of GluN1/GluN2A activated by L -glutamate and analysed by one-way ANOVA with Tukey's post hoc test. Full size image We first evaluated GluN2A–(GluN2D–D1D2) chimeric receptors, which are the GluN2A subunits engineered to contain the entire LBD (that is, both D1 and D2 regions) of GluN2D. The GluN2A–(GluN2D–D1D2) receptors had a slower deactivation time course for L -glutamate ( τ Fast =170±35 ms; τ Slow =740±230 ms; n =5) compared with wild-type GluN1/GluN2A ( n =21; Table 2 ). By contrast, the GluN2A–(GluN2D–D1D2) receptors had a similar time course for D -glutamate ( τ Fast =12±1.9 ms; τ Slow =200±49 ms; n =5; Supplementary Table S3 ) as the wild-type GluN1/GluN2A receptors ( τ Fast =16±1.3 ms; τ Slow =280±130 ms; n =7; Table 1 ). This observation demonstrates that the full LBD can uniquely influence the deactivation time course of GluN1/GluN2D receptors activated by L -glutamate but not D -glutamate. Of note, the GluN2D LBD did not fully interconvert the deactivation time course of GluN2A to that of GluN2D, consistent with the recently suggested role of the ATD in the control of deactivation [20] , [21] . Table 2 GluN2A/2D chimeric and mutant receptors activated by L -glutamate. Full size table We subsequently conducted voltage-clamp recordings of chimeric receptors containing the individual D1 or D2 domains of the GluN2D LBD to dissect the potential contributions of the D1 and D2 regions to the change in L -glutamate deactivation time course. The GluN1/GluN2A–(GluN2D–D1) receptors, which contain the D1 domain of the GluN2D subunit, had slower deactivation time course compared with the wild-type GluN1/GluN2A receptors ( τ Fast =98±4.7 ms; τ Slow =410±56 ms; n =5; Table 2 ). The GluN2A–(GluN2D–D2) receptor, which includes the GluN2D hinge loop region, also deactivated more slowly than wild-type GluN1/GluN2A following the removal of L -glutamate ( τ Fast =110±5.6 ms; τ Slow =660±83 ms; n =7). These data suggest that both the lobes of the LBD influence the deactivation time course of the GluN1/GluN2D NMDA receptors. Because the deactivation time course is related both to agonist unbinding and channel gating, we measured the L -glutamate EC 50 and estimated the open probability ( P Open ) using the rate of onset of MK-801 block following activation by L -glutamate and glycine [38] for chimeric NMDA receptors expressed in Xenopus oocytes. The estimated P Open values of the chimeric receptors were not significantly different from that of the wild-type GluN2A ( Supplementary Table S4 ), consistent with previous studies showing that the ATD is the primary determinant of the P Open of both GluN2A and GluN2D [21] . Both GluN2A–(GluN2D–D1) and GluN2A–(GluN2D–D2) had lower EC 50 values for L -glutamate (EC 50 =0.68±0.20; n =4 and EC 50 =1.2±0.20; n =4, respectively) compared with GluN2A ( Table 2 ). The potency of L -glutamate in the GluN2A–(GluN2D–D1D2) receptors (EC 50 =0.44±0.082; n =6) was identical to the wild-type GluN2D NMDA receptors (EC 50 =0.48±0.078; n =4), in contrast to deactivation time course, which is shifted only partially towards the value for wild-type GluN2A ( Table 2 ). The crystal structures show that the hinge within D2 of the LBD is the most structurally divergent region between the GluN2A and GluN2D LBDs, and is subjected to ligand-specific conformational changes. Using the GluN2A and GluN2D LBD structures as a guide, we identified two residues that varied between the GluN2A and GluN2D hinge regions. We evaluated whether we could transfer the slower time course of GluN2A–(GluN2D–D2) chimeric receptors to GluN2A receptors by exchanging individual residues within the structurally divergent hinge. Consistent with data from chimeric receptors, GluN2A-Y754K deactivated with a slower time course for L -glutamate ( τ Fast =110±7.5 ms; τ Slow =950±150 ms; n =20; Table 2 ) and a slower deactivation time course for D -glutamate ( τ Fast =27±1.4 ms; τ Slow =400±130 ms; n =8; Supplementary Table S5 ) compared with wild-type GluN2A. By contrast, exchanging both divergent residues in GluN2A did not significantly alter deactivation time course ( Table 2 ). Furthermore, the reverse experiment of moving the divergent residues in the GluN2A hinge region into GluN2D does not accelerate the deactivation; rather, it either has no effect or causes a significant lengthening of deactivation compared with wild-type GluN2D ( Table 2 , Supplementary Table S5 ). These data show that the structurally divergent region, while capable of influencing deactivation, by itself cannot fully account for differences in deactivation rates observed in the GluN2A–(GluN2D–D2) chimeric receptors. This is consistent with the idea that the structural determinants of deactivation within these multimeric receptors are complex, and may involve parts of the LBD outside the hinge region and perhaps in parts of receptor not included in the crystal structures studied here. One of the remarkable characteristics of NMDA receptors is the large difference in the deactivation rate among NMDA receptors containing different GluN2 subunits, with the most prominent difference occurring between GluN2A- and GluN2D-containing receptors. An exceptionally slow rate of deactivation is a hallmark of the GluN1/GluN2D NMDA receptors and may be important for early brain development. Here we show that L -glutamate, but not other linear agonists, produces both a unique conformation and slow deactivation in GluN1/GluN2D NMDA receptors. The relationship between EC 50 values and deactivation rates involves gating, and thus is complex [39] , [40] , [41] , [42] . For GluN1/GluN2D receptors (but not GluN1/GluN2A receptors), the relative contribution of the fast and slow exponential components describing deactivation varies widely. Furthermore, data from the chimeric GluN1/GluN2A receptors containing the GluN2D LBD suggest that deactivation is dependent on ligand stereochemistry. Variation in ligand structure has long been known to alter deactivation rates of ligand-gated ion channels, first being described in studies of the muscle nicotinic receptor. For example, the deactivation time course of end-plate currents is accelerated by the release of the false neurotransmitter acetylmonoethylcholine, which shows brief channel open time compared with acetylcholine [43] . Similar experiments with D -glutamate in cultured hippocampal neurons also illustrate the dependence of deactivation rate on the activating ligand [44] . Furthermore, multiple studies on native and recombinant NMDA receptors have described an agonist dependence of deactivation rate and single-channel properties, including mean open time and shut-time durations [4] , [19] , [45] , [46] . However, what seem unique about GluN2D are the marked structural changes in the isolated GluN2D LBD when bound to L -glutamate compared with other ligands and the GluN2A LBD. The crystal structure of a full-length tetrameric AMPA receptor has established that the isolated LBDs accurately represent the extracellular domains in the intact receptors [5] . Therefore, although there may be a minor difference in the orientation of the hinge residues between full-length GluN1/GluN2D receptors and the isolated GluN2D LBD, the divergence of this region for L -glutamate compared with other agonists suggests that L -glutamate induces unique intraprotein interactions within GluN2D compared with other linear ligands bound to GluN2D or L -glutamate bound to GluN2A. Accumulating evidence indicates that multiple regions of the GluN2 subunits are involved in regulation of the deactivation time course. Recent studies have shown that the ATD and the 16-amino-acid linker between the ATD and LBD (ATD–D1 linker) control the deactivation rate and open probability. Substitutions of the ATD or ATD–D1 linker from GluN2A with that from GluN2D result in approximately a sixfold or twofold increase in deactivation time course, respectively [20] , [21] . In the current study, we show that the substitution of the LBD of GluN2A with that of GluN2D also slows the deactivation time course for L -glutamate to a similar degree as the ATD substitution ( Table 1 ). Evaluation of individual domains D1 and D2, as well as individual residues in the hinge region, suggests that the structural determinants of deactivation within the LBD are broadly distributed. Thus, in addition to the ATD, we propose that the LBD is also an important determinant of the deactivation process for L -glutamate [33] , [47] . Remarkably, the GluN2D LBD does not control the deactivation time course of D -glutamate-induced currents, indicating that the LBD of GluN2D may distinctively sense L -glutamate from other linear ligands. Previous studies of glutamate receptor LBDs have indicated that opening and closing of the bilobed clamshell structure on ligand binding and unbinding translate into the major physical driving force for gating of ion channel pores [7] , [48] , [49] . The crystallographic analyses conducted here show that the extent of domain closure between D1 and D2 in the GluN2D LBD structures is nearly identical when complexed with the four linear ligands ( L - and D -glutamate, L -aspartate and NMDA). However, a substantial difference in conformation is observed in the region containing the hinge loop at the backside of the ligand-binding site, including helix-D, -E, and -F, and loop-D in D2 between the structures in complex with L -glutamate and other ligands. The conformation of the hinge loop in the L -glutamate-bound form is such that the residues can no longer interact with helix-D and loop-D, making them highly disordered or flexible. It is plausible that this change in helix-D and loop-D orientation can affect gating properties (and thus deactivation time course) because they are in proximity to the region at which transmembrane helices are tethered in the intact receptors. The hinge region may also be important for sensing L -glutamate, even though it is not directly involved in binding, because deactivation rates of D -glutamate-induced currents are not changed in the chimeric or mutant receptors for which this region is altered. In the GluN1 subunit, a similar site is important for discriminating partial agonists from full agonists [10] . The equivalent structural motifs involving the hinge loop (strand 14 in GluN1) and helix-E and -F (helix-F and -G in GluN1) in GluN1 LBD have conformational variability between the glycine-bound and partial agonist-bound forms, thereby serving as a sensor for discriminating types of ligands and regulating the open probability of the ion channel. Molecular biology cDNAs for the recombinant rat wild-type NMDA receptor subunits GluN1-1a (GenBank U11418, U08261; hereafter GluN1), GluN2A (GenBank D13211) and GluN2D (GenBank L31611) were used for recordings. Constructs encoding chimeric rat GluN2A and GluN2D proteins for GluN2A–(GluN2D–D1D2), GluN2A–(GluN2D–D1) GluN2A–(GluN2D–D2) and point mutants were developed, as previously described [21] , [47] . All receptors were verified by DNA sequencing and were subcloned into the pCI-neo vector, except GluN2A (wild type; pcDNA1/AMP vector). Amino-acid composition of chimeric receptors is given in Supplementary Table S6 . Two-electrode voltage-clamp recordings Preparation and injection of antisense RNAs into Xenopus laevis oocytes as well as all two-electrode voltage-clamp recordings ( V Hold =−30 to −60 mV) were performed, as previously described [50] . Oocytes were stored at 15 °C in Barth's culture bath containing 88-mM NaCl, 5-mM Tris-HCl, 2.4-mM NaHCO 3 , 1-mM KCl, 0.82-mM MgSO 4 , 0.41-mM CaCl 2 and 0.33-mM Ca(NO 3 ) 2 at pH 7.4. Oocytes were injected with 5–10 ng of antisense RNAs synthesized in vitro from linearized template cDNA at a ratio of 1 GluN1 subunit to 2 GluN2 subunits. Recordings were made 2–4 days before injection at 23 °C (room temperature). The external bath solution contained 90-mM NaCl, 10-mM HEPES, 1-mM KCl, 0.5-mM BaCl 2 and 0.01-mM EDTA at pH 7.4. Voltage electrodes were filled with 0.3-M KCl, and current electrodes contained 3-M KCl. Voltage and data acquisition were controlled with a two-electrode voltage-clamp amplifier (OC725, Warner Instruments), and an eight-modular valve positioner (Digital MVP Valve)-controlled solution exchange. Recording solutions were prepared in external bath solution and contained glycine (30 μM) and glutamate (0.1–100 μM). MK-801 (200 nM; Sigma-Aldrich) was prepared in bath solution containing glutamate (100 μM) and glycine (30 μM). Cell culture Human embryonic kidney-293 cell lines (CRL 1573; ATCC; hereafter HEK cells) were plated on 5-mm diameter glass coverslips (Warner Instruments) coated in 100-μg/ml poly- D -lysine and were maintained in 5% humidified CO 2 at 37 °C in DMEM (cat. no. 11960; Invitrogen) supplemented with 10% fetal bovine serum, 10 U per ml penicillin and 10 μg per ml streptomycin. HEK cells were transiently transfected using Fugene6 (Roche Diagnostics) with cDNA encoding green fluorescent protein, GluN1, and GluN2A, GluN2D, or a mutant or chimeric GluN2 subunit at a ratio of 1:1:1 for 0.5 μg per well total cDNA [21] . Following transfection, cells were incubated in media supplemented with NMDA receptor antagonists D , L -2-amino-5-phosphonovalerate (200 μM) and 7-chlorokynurenic acid (200 μM). Whole-cell voltage-clamp recordings Voltage-clamp current recordings ( V Hold =−60 mV) were conducted on HEK cells using an Axopatch 200B amplifier (Molecular Devices) and digitized by Axon pClamp10 software. Recordings were filtered at 8 kHz using an eight-pole Bessel filter (−3 dB; Frequency Devices) and digitized at 40 kHz. Thin-walled borosilicate glass (Warner Instruments, 1.5 mm/1.12 mm outer diametre/inner diametre, cat. no. TW-150F-4) was used to form recording micropipettes, which were filled with an internal solution containing 110-mM D -gluconate, 110-mM CsOH, 30-mM CsCl, 5-mM HEPES, 4-mM NaCl, 0.5-mM CaCl 2 , 2-mM MgCl 2 , 5-mM BAPTA, 2-mM NaATP and 0.3 NaGTP (pH 7.35). Cells were bathed at 23 °C in external solution that contained 150-mM NaCl, 10-mM HEPES, 30-mM D -mannitol, 3-mM KCl, 0.5-mM CaCl 2 and 0.01-mM EDTA at pH 8.0. Macroscopic currents were evoked from cells lifted into the path of a two-barrel theta tube by application of 0.05-mM glycine, followed by 1-s pulses of agonist solutions containing 0.05-mM glycine plus 0.1–1 mM of L -glutamate or other GluN2 ligands, and returned to the initial 0.05-mM glycine application for 3–25 s. In paired-pulse experiments, GluN1/GluN2D receptors were activated by 2-ms or 4-s pulses of 1-mM L -glutamate and 0.05-mM glycine, followed by a second pulse applied 2–10 s after the removal of the first pulse for 2 ms or 4 s. Rapid solution exchange for macroscopic recordings was accomplished with a theta pipette controlled by a piezoelectric translator (Burleigh Instruments). Whole-cell 10–90% solution exchange times were ~4 ms and were determined, as previously described [51] , and 10–90% open-tip solution exchange times were under 0.5 ms. Between 5 and 10 sweeps were recorded for each condition. Data analysis For each macroscopic current condition, the current response waveforms recorded under voltage clamp were aligned on the point of steepest rise and averaged following subtraction of the preapplication baseline. Current amplitude, 10–90% rise time and deactivation time constant were determined. Relative maximum response was determined by expressing the response of a maximally effective concentration of a given agonist as a percentage of the response to 1-mM L -glutamate recorded in the same cell. The deactivation time constant was fit using the following equation: where τ Fast is the fast deactivation time constant, τ Slow is the slow deactivation time constant, Amp Fast is the amplitude of the fast deactivation component, Amp Slow is the amplitude of the slow deactivation component and t =0 is defined as the peak of the response at the moment deactivation is initiated. Weighted deactivation time constants ( τ W ) were determined using the following equation: Relative P Open was estimated for chimeric receptors and point mutants by analyzing the time course for the onset of MK-801 inhibition, as previously described [38] . Briefly, the rate of onset of MK-801 inhibition was calculated using the following equation: where τ MK-801 block is the time constant for the onset of MK-801 block. τ MK-801 block was calculated using the single-exponential equation where Amp is the amplitude of the current response and steady state describes the steady-state current observed in the presence of incomplete MK801 block. Open probability ( P Open ) for the chimeric receptors and point mutants were calculated from the wild-type receptor open probability and the block rate of MK-801 using the following equation where GluN2A P Open was 0.48 and GluN2D P Open was 0.012, determined from single-channel data [21] . Concentration–response curves were fitted for each oocyte with the Hill equation where EC 50 is the agonist concentration that produces a half-maximal effect, and n H is the Hill coefficient. The responses of gating models were evaluated by numerical integration (Channelab, Synaptosoft) and assessment of the Q matrix [13] to determine the deactivation time course and EC 50 values as a function of the agonist dissociation rates (SCALCS, HJCFIT, kindly provided by Dr David Colquhoun, University College London). Three models were adapted as shown in Supplementary Figure S1 to simulate NMDA receptor responses. Data are reported as mean±s.e.m. and were evaluated statistically using one-way ANOVA and Tukey's post hoc test. Significance for all tests was set at P <0.05. EC 50 values are reported as mean±s.e.m., but statistical analyses were performed on the log(EC 50 ), as EC 50 demonstrates a lognormal distribution [52] . Protein purification and crystallization The GluN2D LBD construct used in this structural study was defined as Asp424–Arg564 and Thr686–Asn827 connected by a Gly–Thr linker. The GluN2D LBD protein was expressed as a fusion protein to small ubiquitin-like modifier (SUMO) with the N-terminal hexa-histidine tag in Origami B (DE3) strain (Novagen) under T7 promoter in pET22b(+) (Novagen). After growing cells to OD 600 =4 in a fermenter (BioFlo3000; New Brunswick) at 37 °C, protein expression was induced by 0.5-mM IPTG at 15 °C for 36 h. The GluN2D LBD proteins were purified using Nickel-chelating Sepharose (GE Healthcare) and digested by ubiquitin ligase protease-1 to remove SUMO. The sample was further purified by a combination of Q-Sepharose, SP-Sepharose and Superdex200 (GE Healthcare). Structural studies The purified GluN2D LBD proteins were concentrated to ~5 mg ml −1 and dialyzed against a buffer containing 10-mM Tris-HCl (pH 8), 50-mM NaCl and 10 mM of D - and L -glutamate, L -aspartate or NMDA. All of the crystals were produced by vapour diffusion at 17 °C in hanging drops containing 2:1 protein to reservoir solution composed of 3.5- to 4.5-M sodium formate, 100-mM CAPS (pH 9–10) and 8–12% of 1,4-butanediol. The concentration of 1,4-butanediol was raised to 14% for cryoprotection of the crystals during data collection. The X-ray diffraction data was collected at X25, X26C and X29 beamlines at the National Synchrotron Light Source at Brookhaven National Laboratory and processed using HKL2000. The structure of the L -glutamate-bound form was determined by molecular replacement using an alanine chain of the GluN2A LBD structure (PDB code: 2A5S ) as a molecular search probe and by using the program Phaser [53] . The GluN2D LBD structures in complex with L -aspartate, D -glutamate and NMDA were determined by molecular replacement using the structure of GluN2D LBD in complex with L -glutamate. Structural refinement and model building were performed with PHENIX [54] and Coot [55] , respectively. Accession codes: Coordinates for GluN2D LBD structures in complex with D - and L -glutamate, L -aspartate and NMDA have been deposited in the Protein Data Bank with accession codes 3OEL , 3OEN , 3OEK and 3OEM , respectively. How to cite this article: Vance, K. M. et al . Ligand-specific deactivation time course of GluN1/GluN2D NMDA receptors. Nat. Commun. 2:294 doi: 10.1038/ncomms1295 (2011).